Selecting core-hole localization or delocalization in CS2by photofragmentation dynamics Electronic core levels in molecules are highly localized around one atomic site. However, in single-photon ionization of symmetric molecules, the question of core-hole localization versus delocalization over two equivalent atoms has long been debated as the answer lies at the heart of quantum mechanics. Here, using a joint experimental and theoretical study of core-ionized carbon disulfide (CS 2 ), we demonstrate that it is possible to experimentally select distinct molecular-fragmentation pathways in which the core hole can be considered as either localized on one sulfur atom or delocalized between two indistinguishable sulfur atoms. This feat is accomplished by measuring photoelectron angular distributions within the frame of the molecule, directly probing entanglement or disentanglement of quantum pathways as a function of how the molecule dissociates. Schrödinger’s cat is an iconic symbol of a famous thought experiment in quantum mechanics. The original version [1] refers to a cat trapped unseen inside a chamber connected to a Geiger counter monitoring a radioactive sample. If, and only if, the counter detects a signal, cyanide gas is released in the chamber, killing the cat. In Schrödinger’s gedanken experiment, the probability of a signal is exactly 50%, and one does not know a priori whether the cat lives or dies until the chamber is opened. Before this, two states of equal probability (living cat versus dead cat) are entangled, and the quantum depiction of the system is represented by their equal superposition. Schrödinger saw this as a paradox in the interpretation of quantum systems. In the present work, a molecular equivalent to this thought experiment is studied experimentally. The two states of equal probability are created by ionization of a core level in a symmetric molecule (photoionization of a S 1 s electron from carbon disulfide, CS 2 , in which the sulfur atoms are chemically equivalent). Subsequent to photoionization, the molecule usually fragments into many ions and free electrons. Using multi-coincidence measurements of several of these charged particles, it is possible to determine the process by which the molecule dissociates. As we show, in some cases a specific fragmentation pattern indicates which sulfur atom was initially ionized, and the experiment disentangles the quantum states. In the jargon of the field, the core hole is ‘localized’ (and the cat, for example, is found to be alive). In contrast, other fragmentation patterns cannot distinguish between the sulfur atoms, the core hole is ‘delocalized’, and the quantum states remain entangled and indistinguishable (by analogy, the chamber is never opened). Other studies of ionization of equivalent core levels in symmetric molecules have focused on a number of issues regarding core-hole localization and symmetry-breaking, all tied to the peculiar nature of the quantum-mechanical description [2] , [3] , [4] , [5] , [6] , [7] , [8] . Observations of Doppler-like energy shifts have also been considered as manifestations of core-hole localization in the photoionization of O 2 in first-step Auger decay [9] and in secondary Auger decay [10] . In general, the scheme used to probe localization versus delocalization has been to break the symmetry of highly symmetric molecular systems. Substituting one 14 N atom by 15 N in N 2 (ref. 11 ), Rolles et al . succeeded in detecting a small isotope effect in the vibrationally resolved N 1 s photoelectron spectra attributed to symmetry breaking and partial core-hole localization induced by non-Born-Oppenheimer coupling. Using molecular-frame photoelectron angular distributions (MFPADs) as a probe, while no asymmetry was observed in N 2 (ref. 12 ), a very slight one was observed in CO 2 , both in C 1 s (ref. 13 ) and in O 1 s (refs 14 , 15 ) photoionizations. The latter has been attributed to a degree of core localization due to asymmetric vibration, competing with the Auger decay [14] , [16] . In this study, we investigate the conditions in which core-hole localization or delocalization can be observed through the different mechanisms leading to three-body fragmentation of a symmetric triatomic molecule, namely carbon disulfide, CS 2 . We show that a multi-coincidence measurement is able to probe either the localization or the delocalization of a core hole in the same well-defined quantum state, by monitoring the different (and complex) ways in which the core-ionized molecule fragments. This selectivity is accomplished by measuring MFPADs in which multiple ions and the photoelectron are detected from individual molecular-fragmentation events after deep-core-level photoionization of a S 1 s electron. The advantage offered by initially ionizing S 1 s is that the ultimate degree of ionization, after Auger decay, is typically +4, offering a richer array of possible fragmentation pathways originating from the photoionized state. Sulfur 1 s core ionization of carbon disulfide In CS 2 , the chemical equivalence of the two sulfur atoms translates into the energetic indistinguishability of the two S 1 s core levels, 1 s L and 1 s R. An equivalent description is to consider their symmetric and antisymmetric combinations, g and u, which are delocalized over the two atoms and too close in energy to be resolved. Because of the large internuclear distance between the two S atoms (~6 a.u. ), the two 1 σ g and 1 σ u states are nearly completely degenerate (<1 meV, according to our Hartree-Fock calculations), while the lifetime broadening of the S 1 s core hole is 520 meV (ref. 17 ). The incoherent sum of electron emission from both orbitals is therefore recorded, and the two descriptions (1 σ g+1 σ u) and (1 s L+1 s R) are completely equivalent and both can be employed on the same footing for further analysis. The binding energy of the S 1 s core electrons in CS 2 is 2,478 eV (ref. 18 ). Core ionization leaves the system in a highly unstable state that decays either through photon emission or Auger decay, the latter being the dominant channel (~90%). After deep-core ionization, relaxation processes often occur in a cascade involving multiple Auger decays, several electrons are emitted sequentially, and highly charged ions are produced [18] , [19] , [20] . When a molecule containing only a few atoms is multiply ionized and left in a charge state in which each constituent atom can carry positive charge, it primarily dissociates through Coulomb repulsion. Deep-shell ionization can thus lead to the production of a large variety of fragment ions representing complex fragmentation pathways. The main decay of CS 2 after S 1 s photoionization is the three-body fragmentation of into S + + C + + S 2+ (36.3±1.6% of all fragments) [18] , [21] , [22] . As it turns out, following the path from ionization of a S 1 s core electron in CS 2 to the production of two distinguishable sulfur ions, S + and S 2+ provides an ideal experimental scheme to study core-hole localization versus delocalization. To begin, consider the process depicted in Fig. 1 , in which the decay of created after S 1 s photoionization is used as a specific example that is no doubt typical of many other systems. Starting from a core-ionized CS 2 + molecule (top), it is not known a priori on which sulfur atom the core hole is created (1 s L or 1 s R). Different pathways can lead to S + + C + + S 2+ (bottom). Because parity is conserved in electromagnetic interactions, the final state of the ions can be treated as a symmetric superposition of the situations in which S 2+ is detected either to the right or to the left along the molecular axis. Ultimately, experimental detection of an ion forces the final state to collapse, revealing one of these two situations. In the scheme in Fig. 1 , S 2+ is arbitrarily detected to the right, providing a frame of reference for the dissociation process. Starting from a S 1 s hole with a lifetime of about 1 fs, it is realistic to consider that the ultrafast electronic decay involves an initial KLL Auger decay on the same sulfur atom, followed by charge redistribution and asymmetric fragmentation associated with the initial site of the core hole. Still, the overall process (L+R) is strictly symmetrical, and a multitude of electronic decay processes is available, leading either to a symmetrical multiply ionized cation before dissociation, or to an asymmetrical charge distribution specific to the initial core-hole site. But, even in the latter case, subsequent fragmentation may only partially favour one dissociative channel over its mirror image [14] . If, in addition, the experiment detects the photoelectron in coincidence with the ions, it is possible to measure MFPADs, providing a detailed look at the ionization/fragmentation process. 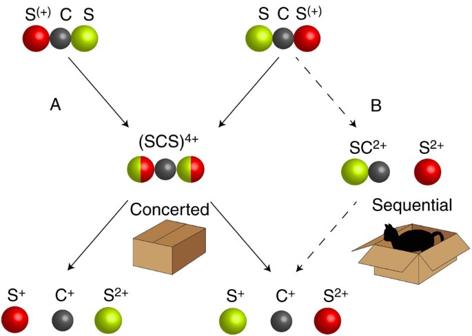Figure 1: Schematic representation of the core-hole decay and molecular-fragmentation processes. Top:ions created by S 1sphotoionization of CS2at 2,488 eV photon energy. The site of the initial S 1score hole is indicated in red (left, 1sL; right, 1sR). Middle: intermediate multiply charged cations created by Auger decay of the S 1score hole. On the left is aion produced when charge transfer is faster than molecular fragmentation. On the right, fragmentation competes with charge transfer, leading to a partially fragmented intermediate state. Bottom: final fully fragmented state, with the S2+ion detected to the right. The final state is reached in two distinct ways: (1) concerted fragmentation of(Case A, solid arrows), which leads to the formation of S++C++S2+with equal decay probabilities from 1sL and 1sR; or (2) sequential fragmentation of the molecule (Case B, dashed arrows), in which only the 1sR core hole is associated with the S2+fragment. The opened and unopened boxes (chambers) refer to the analogy to Schrödinger’s cat discussed in the text. Figure 1: Schematic representation of the core-hole decay and molecular-fragmentation processes. Top: ions created by S 1 s photoionization of CS 2 at 2,488 eV photon energy. The site of the initial S 1 s core hole is indicated in red (left, 1 s L; right, 1 s R). Middle: intermediate multiply charged cations created by Auger decay of the S 1 s core hole. On the left is a ion produced when charge transfer is faster than molecular fragmentation. On the right, fragmentation competes with charge transfer, leading to a partially fragmented intermediate state. Bottom: final fully fragmented state, with the S 2+ ion detected to the right. The final state is reached in two distinct ways: (1) concerted fragmentation of (Case A, solid arrows), which leads to the formation of S + +C + +S 2+ with equal decay probabilities from 1 s L and 1 s R; or (2) sequential fragmentation of the molecule (Case B, dashed arrows), in which only the 1 s R core hole is associated with the S 2+ fragment. The opened and unopened boxes (chambers) refer to the analogy to Schrödinger’s cat discussed in the text. Full size image Figure 1 properly distinguishes between two different decay paths that depend on the occurrence of charge transfer in the ion before dissociation. In case A, represented by solid lines, Auger decay leads to a symmetrically charged cation, with equal decay probabilities from 1 s L and 1 s R and equal fragmentation probabilities to S + +C + +S 2+ . For case A to be observed, charge redistribution must occur faster than molecular fragmentation, and the dissociation must be concerted, that is, the three atomic cations are ejected simultaneously in a Coulomb explosion. As a result, information on the initial core hole is lost, and one cannot tell from S + or S 2+ where the initial core ionization occurred; the photoionization process can only be described by a superposition of states (1 s L+1 s R) in a delocalized picture. In analogy with Schrödinger’s cat, case A corresponds to a situation where the box remains unopened, and the status of the cat is never determined by observation; the observed MFPAD will be completely symmetrical [11] . In case B, represented by dotted lines in Fig. 1 , the molecular ion dissociates before charge transfer occurs; the fragmentation is sequential and asymmetrical, leading to the formation of SC 2+ +S 2+ and eventually to S + +C + +S 2+ . As a result, S 2+ is associated with a 1 s R initial core hole, and the photoionization process is best described in a localized core-hole picture, corresponding to opening the box and observing the status of the cat; the observed MFPAD is expected to be asymmetrical. Because both decay modes A and B occur in CS 2 , the R fragmentation channel is expected to be partially asymmetrical, with 1 s R ionization contributing more than 1 s L ionization. Moreover, because these decay modes can be distinguished kinematically due to their different fragmentation dynamics, it is possible to focus on events that are either totally symmetrical (case A, concerted fragmentation) or very asymmetrical (case B, sequential fragmentation). The remainder of this paper demonstrates under what conditions case A or case B may be observed experimentally, providing a new way to probe core-hole localization versus delocalization. Disentanglement of the fragmentation mechanisms All of the coincidence measurements described in this article were performed at 2,488 eV photon energy, 10 eV above the sulfur 1 s ionization threshold, focusing on the three-body fragmentation channel depicted in Fig. 1 . Experimental details can be found elsewhere [23] . Convenient visualizations of three-body fragmentation dynamics are provided by Dalitz plots and Newton diagrams. These two representations are shown in Fig. 2 . The Dalitz plot [24] in Fig. 2a is constructed using the normalized coordinates ε i =| P i | 2 /∑ i | P i | 2 for each ion i of momentum P i and the Cartesian coordinates and y D = ε 1 −1/3. This probability plot shows the momentum correlation among the three fragment ions. Momentum conservation requires that all events lie inside a circle, and for each ion the distance from the opposite side of the regular triangle is ε i . Two distinct contributions are observed, corresponding to different dissociation mechanisms. The main contribution near coordinate corresponds to simultaneous ejection of the three ions via concerted fragmentation (case A, Fig. 1 ). The linear ground-state geometry of the molecule is reflected in the energy distribution of C + . Because the carbon atom is located at the centre of the molecule between the two sulfur atoms, it acquires little kinetic energy when the fragmentation process is simultaneous. A second weaker contribution in the Dalitz plot appears slightly above and to the right of the main contribution. It corresponds to sequential fragmentation (case B, Fig. 1 ) in which first dissociates into S 2+ and CS 2+ , after which CS 2+ further dissociates into S + and C + . As a result, the distribution reflects momentum sharing between S 2+ and the temporarily undissociated CS 2+ fragment. 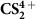Figure 2: Fragmentation dynamics of. (a) Dalitz plot of thethree-body fragmentation pattern. (b) Newton diagram showing the momentum vectors of C+and S+with respect to the momentum of S2+(red arrow). Figure 2: Fragmentation dynamics of . ( a ) Dalitz plot of the three-body fragmentation pattern. ( b ) Newton diagram showing the momentum vectors of C + and S + with respect to the momentum of S 2+ (red arrow). Full size image The Newton diagram in Fig. 2b shows relative momentum distributions of S + , C + and S 2+ , with the centre of mass of the three ions defining the origin. Newton diagrams provide a direct image of dissociation dynamics in the molecular frame, with the origin being the position of the undissociated molecule. To construct this diagram, the direction of S 2+ was fixed (red arrow, P y =0) to provide a frame of reference for the momenta of C + and S + . Furthermore, the momenta for C + are plotted only in the upper half plane ( P y >0) and those for S + only in the lower half plane ( P y <0). The main contribution, due to concerted fragmentation, produces momenta of C + and S + along the mean directions indicated by the black and blue arrows in Fig. 2b . The C + fragment is not emitted perpendicular to the molecular axis, but at a mean angle of 114° with respect to S 2+ , in part because it experiences a stronger Coulomb repulsion from S 2+ on one side than from S + on the other side. Most likely, C + also gains momentum from a slight bending of the ionized molecule due to vibrational motion, and the Coulomb repulsion exaggerates the bent geometry of the molecule in the momentum distribution. The contribution due to sequential fragmentation can be seen more clearly in the Newton diagram. The C + and S + fragments are emitted in opposite directions and their momenta are distributed around a circle, illustrating that the intermediate CS 2+ ion acquires some angular momentum and has time to rotate with respect to S 2+ before it dissociates. We note that, in the concerted case, the momentum distribution of C + spreads from 10 to 150 a.u., while in the sequential case, C + has a very narrow momentum distribution (±10 a.u.) centred around 80 a.u. Therefore, the two mechanisms can be disentangled based on momentum, or as explained below, kinetic-energy discrimination. Similar observations regarding competition between concerted and sequential fragmentation were made previously with regard to dissociation of CO 2 after C 1 s photoionization, including rotation of the undissociated CO 2+ fragment [25] , [26] . Neumann et al . observed that the two different fragmentation pathways correspond to different kinetic-energy releases and can be separated by selecting a proper kinetic-energy range [25] . In the present case, concerted and sequential fragmentation of CS 2 can be separated by filtering the events with the kinetic energy of the S + ion, as shown in Fig. 3 . The same clear separation is observed in filtered Dalitz plots (not shown). The S + ions with higher kinetic energies, from 6 to 25 eV, correspond to a kinetic-energy distribution of S 2+ centred around 14 eV and a distribution of C + centred around 5 eV. These distributions are associated with concerted fragmentation, as illustrated by the Newton diagram in Fig. 3c . Only the main contribution of C + ions emitted near 114° relative to the S 2+ ion is apparent. In contrast, S + ions with lower kinetic energies, from 0 to 6 eV, correspond to kinetic-energy distributions of both S 2+ and C + centred around 10 eV. For these events, C + ions gain more kinetic energy, and their momenta are distributed on a circle displaced by 60 a.u. relative to the centre of mass. The Newton diagram in Fig. 3b exhibits only half of this circle because, for clarity, these coincidence data have been filtered further by selecting only the low kinetic-energy S + ions moving in the same direction as S 2+ . As a result, only C + fragments moving away from S 2+ are visible in Fig. 3b . This Newton diagram illustrates that undissociated CS 2+ ions rotate with respect to S 2+ before they dissociate, a clear footprint of sequential fragmentation. The existence of predissociative states of CS 2+ with lifetimes long enough to allow for this rotation is supported by previous configuration–interaction potential-energy calculations [27] , which show that the potential-energy curves of CS 2+ have a shallow minimum, with a lifetime estimated to be 10 ps< τ ≪ 1 μs (ref. 28 ). 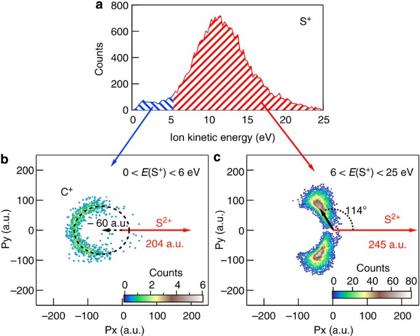Figure 3: Selection of the fragmentation pathway. Top: (a) kinetic-energy distribution of the S+fragment in the three-body fragmentation of CS2following S 1sphotoionization. Bottom: Newton diagrams showing momentum distributions of the C+fragment with respect to a fixed direction of the S2+ion (red arrows in (b) and (c)). (b) Newton diagram associated with low kinetic-energy S+ions (0<E(S+)<6 eV). (c) Newton diagram associated with high kinetic-energy S+ions (6<E(S+)<25 eV). Figure 3: Selection of the fragmentation pathway. Top: ( a ) kinetic-energy distribution of the S + fragment in the three-body fragmentation of CS 2 following S 1 s photoionization. Bottom: Newton diagrams showing momentum distributions of the C + fragment with respect to a fixed direction of the S 2+ ion (red arrows in ( b ) and ( c )). ( b ) Newton diagram associated with low kinetic-energy S + ions (0< E (S + )<6 eV). ( c ) Newton diagram associated with high kinetic-energy S + ions (6< E (S + )<25 eV). Full size image Molecular frame photoelectron angular distributions The Newton and Dalitz diagrams in Figs 2 and 3 depicting fragmentation of CS 2 into S + + C + + S 2+ demonstrate that the current experiment can readily distinguish between concerted-dissociation events and sequential-dissociation events. To probe the localized versus delocalized nature of the photoionization process, it is necessary to view the MFPADs associated with each dissociative pathway. To do this, the direction of S 2+ is again taken as a reference to define the orientation of the molecular axis and thus the recoil frame. Because the CS 2+ fragment rotates when dissociation is sequential, information on its initial orientation is lost. Under these circumstances, the ‘molecular frame’ is reduced to the recoil direction of the S 2+ fragment, and the corresponding MFPADs are more correctly described as recoil-frame angular distributions [29] . Nevertheless, MFPADs associated with concerted and sequential fragmentation are shown in Fig. 4 for two orientations of the molecular axis with respect to the polarization vector of the incident radiation, together with theoretical calculations assuming either a localized or a delocalized core hole, as appropriate. 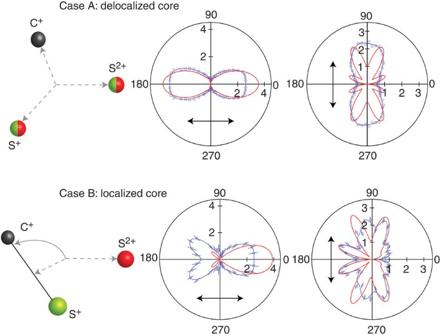Figure 4: Polar plots of molecular-frame photoelectron angular distributions obtained after photoionization of CS210 eV above the S 1sthreshold. Top: MFPADs for concerted fragmentation (Case A), for which a delocalized core-hole picture is the best. Bottom: MFPADs for sequential fragmentation (Case B), for which a localized-core-hole picture is best. In each case, MFPADs are shown for the molecular axis oriented either parallel or perpendicular to the polarization vector of the incident radiation (black arrows). For the polar plots, S2+is always detected to the right (0°), and the experimental data are shown as blue circles with statistical error bars and a blue curve to guide the eye. Corresponding theoretical calculations are shown as red curves. Figure 4: Polar plots of molecular-frame photoelectron angular distributions obtained after photoionization of CS 2 10 eV above the S 1 s threshold. Top: MFPADs for concerted fragmentation (Case A), for which a delocalized core-hole picture is the best. Bottom: MFPADs for sequential fragmentation (Case B), for which a localized-core-hole picture is best. In each case, MFPADs are shown for the molecular axis oriented either parallel or perpendicular to the polarization vector of the incident radiation (black arrows). For the polar plots, S 2+ is always detected to the right (0°), and the experimental data are shown as blue circles with statistical error bars and a blue curve to guide the eye. Corresponding theoretical calculations are shown as red curves. Full size image The MFPAD measurements beautifully demonstrate the experimental scheme depicted in Fig. 1 . In case A (concerted fragmentation), the MFPADs for both molecular orientations are symmetrical with respect to the plane of symmetry of the molecule (S 2+ to the right, S + to the left). Exactly the same characteristics are observed in calculations assuming a delocalized core hole. Therefore, MFPADs measured in this case are insensitive to which sulfur atom is ionized (that is, 1 s L or 1 s R), and localization of the core hole is not feasible for these events. It is likely that rapid charge transfer occurs before dissociation, and any information on the initial site of the core hole is lost. In case A, the photoionization process has to be treated as delocalized, and the box containing the cat remains unopened. In contrast, for case B (sequential fragmentation), the MFPADs for both molecular orientations are quite asymmetrical with respect to the axis of the molecule, and the main structures agree very well with calculations assuming a localized core hole: the MFPDs obtained for parallel and perpendicular molecular orientations show strongly asymmetric angular distributions with respect to the detection direction of S 2+ (R) and S + (L). The observed asymmetry is direct evidence for localization of the initial core hole on the sulfur atom ultimately detected as S 2+ , precisely because the experiment selected events that lead to sequential dissociation. In case B, the photoionization process has to be treated as localized, the box is opened, and the cat is found to be alive. Although the comparison of the measured and calculated MFPADs clearly evidences the two opposite situations, discrepancies between the experiment and the theory are observed. Notably, in the experimental concerted MFPADs, a slight asymmetry is observed towards the S + fragment. As shown previously [14] , asymmetrical vibration can lead to a slight asymmetry in the MFPAD. Also, because the disentanglement of the two fragmentation mechanisms is based solely on kinetic-energy considerations, this selection is imperfect and both mechanisms can still contribute moderately to the resulting MFPADs, adding asymmetry to the concerted MFPADs and symmetry to the sequential ones. Moreover, it is a general observation that theoretical MFPADs show more structures than experimental ones. Limitations of the recoil axis approximation in real experiments and inherent approximations in the theory are usual causes of discrepancy (see discussion in ref. 30 ). This article has addressed the long-debated question of core-hole localization in molecules. Using the specific example of the S 1 s photoionization of CS 2 , the present work illustrated an experimental method to identify conditions under which either localization or delocalization of a core hole can be observed, in analogy to the iconic Schrödinger’s cat thought experiment. By selecting the dissociation pathway, the effects of rapid charge redistribution could be enhanced or reduced, thus losing or preserving information on the initial location of the core hole. Localization itself was probed by measuring angular distributions of S 1 s photoelectrons in the frame of the molecule. Two distinct cases were observed: a concerted fragmentation after rapid charge redistribution, for which the photoionization process is best described as delocalized, and a sequential fragmentation occurring in competition with charge redistribution, for which the photoionization process is best described as localized. Competition between charge redistribution and fragmentation in a molecule has important consequences for studies in which the location of photon absorption is crucial. Notably, the notion of site-selective fragmentation induced by core-level photoionization, long discussed with regard to radiation damage (see ref. 31 ), should be re-evaluated in light of rapid charge redistribution in the target molecule. Experimental method The experimental results were obtained by measuring the S 1 s photoelectron in coincidence with all three cations: . As noted in the article, this is the main fragmentation channel following S 1 s ionization, so four-particle coincidences could be measured with good statistics despite the low photoionization cross-section for S 1 s (~0.1 Mb (ref. 32 )). The two sulfur ions bear different charges, +1 and +2, and can be distinguished by their different flight times through a double-momentum spectrometer (described in details in ref. 23 ), which vary as a function of the mass and charge of each fragment. The spectrometer can measure in coincidence the momenta of all charged particles created in a single-ionization event. The experiment was performed at beamline LUCIA of the French national synchrotron source SOLEIL, which provided X-rays with 100% linear polarization during eight-bunch operation of the storage ring. The 99%-pure carbon disulfide sample was obtained commercially from Sigma Aldrich. Expansion of the gas (400 mbar) into the interaction chamber (10 −6 mbar) through a 100-μm nozzle produced a cold supersonic jet that was collimated by a 500-μm skimmer before intersecting the photon beam at the focal point of a double momentum spectrometer. An electric field of 140 V cm −1 was used to extract all cations with kinetic energies <30 eV, providing a full 4 π collection angle. Momentum vectors of each particle detected in coincidence are derived from impact positions on the position-sensitive detector and flight times measured with respect to the bunch marker from SOLEIL. Data for each ionization event can be filtered off-line to isolate signal from only the coldest portion of the supersonic molecular beam, as well as to focus on specific ranges of flight time, impact position and/or kinetic energy of a particle. Theoretical calculations The theoretical MFPADS were obtained from accurate solutions of the relevant scattering equations, employing an LCAO multicenter program [33] , [34] , [35] that deals effectively with deep core holes. The code provides transition dipole moments between initial orbitals (1 σ g , 1 σ u , or S 1 s in the localized description) and final continuum orbitals, where an exchange correlation potential has been employed to yield the correct asymptotic Coulomb tail. From these transition dipoles, MFPADS are then computed according to standard formulae [36] , [37] . How to cite this article : Guillemin, R. et al . Selecting core-hole localization or delocalization in CS 2 by photofragmentation dynamics. Nat. Commun. 6:6166 doi: 10.1038/ncomms7166 (2015).